A lysine-rich motif in the phosphatidylserine receptor PSR-1 mediates recognition and removal of apoptotic cells The conserved phosphatidylserine receptor (PSR) was first identified as a receptor for phosphatidylserine, an ‘eat-me’ signal exposed by apoptotic cells. However, several studies suggest that PSR may also act as an arginine demethylase, a lysyl hydroxylase, or an RNA-binding protein through its N-terminal JmjC domain. How PSR might execute drastically different biochemical activities, and whether they are physiologically significant, remain unclear. Here we report that a lysine-rich motif in the extracellular domain of PSR-1, the Caenorhabditis elegans PSR, mediates specific phosphatidylserine binding in vitro and clearance of apoptotic cells in vivo . This motif also mediates phosphatidylserine-induced oligomerization of PSR-1, suggesting a mechanism by which PSR-1 activates phagocytosis. Mutations in the phosphatidylserine-binding motif, but not in its Fe(II) binding site critical for the JmjC activity, abolish PSR-1 phagocytic function. Moreover, PSR-1 enriches and clusters around apoptotic cells during apoptosis. These results establish that PSR-1 is a conserved, phosphatidylserine-recognizing phagocyte receptor. Clearance of apoptotic cells is an integral part of the apoptotic programme and an important event in tissue remodelling, suppression of inflammation and regulation of immune responses [1] , [2] . During apoptosis, phosphatidylserine (PS), which normally is restricted to the inner leaflet of plasma membrane, is externalized on the surface of the dying cells and serves as an ‘eat-me’ signal to trigger phagocytosis [3] , [4] , [5] , [6] , [7] , [8] . Importantly, this apoptotic PS externalization process is highly conserved and has been observed in multiple organisms [3] , [4] , [8] , [9] , [10] , [11] , [12] , [13] . How PS is recognized by phagocytes or the identity of the PS receptor, however, is poorly understood and highly controversial [14] . PSR was first identified as a conserved transmembrane protein on phagocytes that mediates phagocytosis of apoptotic cells by binding to externalized PS on the surfaces of apoptotic cells [3] , [15] . Subsequently, a conserved role of PSR in cell clearance has been supported by numerous studies in which the inactivation or knockdown of PSR compromises phagocytosis of apoptotic cells in humans, mice and zebrafish [16] , [17] , [18] , [19] , [20] , [21] , blocks phagocytic removal of growth-disadvantaged cells by neighbouring wild-type cells in Drosophila [22] , and causes a defect in clearance of somatic apoptotic cells or prevents phagocytic removal of living cells with surface-exposed PS in C. elegans [23] , [24] . On the other hand, several studies have failed to detect a defect in clearance of apoptotic cells in PSR-deficient animals or cells [10] , [25] , [26] , [27] . These observations suggest that PSR plays either a dispensable or a redundant role in the clearance of apoptotic cells, which could be difficult to detect. Recently, several studies suggest that a number of other human membrane proteins, including BAI1, TIM4 and stabilin-2, can serve as PS-recognizing receptors to mediate clearance of apoptotic cells [28] , [29] , [30] . However, none of these proteins, except PSR, is conserved evolutionarily, calling into question the true identity of the PS receptor [14] , which is central to apoptotic corpse clearance in diverse organisms. Adding to the puzzle, several studies report somewhat conflicting biochemical analyses of PSR, suggesting that PSR possesses a histone arginine demethylase activity [31] , a lysyl hydroxylase activity [32] or a single-stranded RNA (ssRNA)-binding activity [33] . However, the in vivo relevance of these new and different PSR biochemical activities remains largely unexplored. The Fe(II) binding site at the amino-terminal (N-terminal) JmjC domain of PSR is critical for the demethylase activity and the hydroxylase activity [31] , [32] . It is unknown how PSR binds PS or ssRNA. These studies have raised major questions about the physiological roles of PSR in animals and the in vivo significance of the differing PSR-associated biochemical activities. We address these issues by dissecting the PSR-1 protein in C. elegans to determine its PS-binding domain and to define the importance of the PS-binding activity to its in vivo function. We find that a unique and conserved lysine-rich motif in the extracellular domain of PSR-1 is critical for PS binding in vitro and clearance of apoptotic cells in vivo and that the JmjC-associated biochemical activities are dispensable for the phagocytic function of PSR-1. In addition to playing a role in clearance of somatic apoptotic cells in C. elegans [23] , PSR-1 is important for clearance of apoptotic germ cells and necrotic cells and similarly acts through the CED-2, CED-5 and CED-12 signalling pathway to promote phagocytosis of dead cells. Consistent with its role as a phagocyte receptor, PSR-1 enriches and clusters around apoptotic cells. These results indicate that PSR-1 is a bona fide PS-recognizing phagocyte receptor important for clearance of both apoptotic and necrotic cells. A short lysine-rich motif in PSR-1 mediates PS binding PSR-1 is predicted to be a type II transmembrane protein [15] , with its N-terminal portion (residues 1–270) inside the cell, its carboxyl-terminal (C-terminal) portion (residues 293–400) extracellular and a short transmembrane domain (residues 271–292) in the middle ( Fig. 1a ). We first tested PS binding by the intra- and extracellular domains of PSR-1. In an in vitro lipid-binding assay, a PSR-1(1–270) maltose-binding protein (MBP) fusion, MBP-PSR-1(1–270), did not bind any phospholipid ( Fig. 1b ), whereas MBP-PSR-1(293–400) or a similar glutathione S -transferase (GST) fusion, GST-PSR-1(293–400), bound PS specifically ( Fig. 1b,c ). These results indicate that the extracellular domain of PSR-1, but not its intracellular domain, binds PS in vitro . 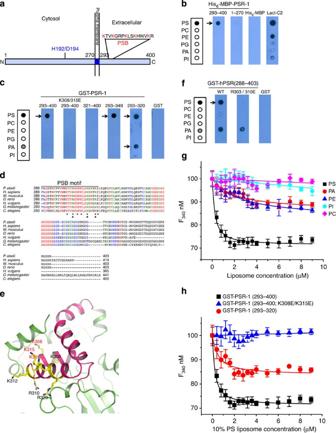Figure 1: Identification of a lysine-rich PS-binding motif in PSR-1. (a) A schematic cartoon of PSR-1 with its extra- and intracellular domains. The conserved Fe(II)-binding site (H192/D194) and the PS-binding motif (PSB) are shown. (b,c,f)In vitrolipid-binding assays. Membrane strips containing equal amounts (500 pmol) of the indicated phospholipids were incubated with 5 μg ml−1of purified proteins as indicated (see Methods). The lactadherin C2 domain (Lact-C2), known to bind PS, is used as a positive control. After washing three times with washing buffer, the membrane strips were probed with anti-His6(b) or anti-GST (c,f) antibodies. PSR-1 domains and mutations included are as indicated. The strip template on the left depicts phospholipids loaded on the membrane. PS, phosphatidylserine; PC, phosphatidylcholine; PE, phosphatidylethanolamine; PG, phosphatidylglycerol; PA, phosphatidic acid; PI, phosphatidylinositol. (d) Sequence alignment of the extracellular domains of PSR proteins from different species. Residues that are identical are indicated in red, residues highly conserved in green, and residues similar in blue. Asterisks indicate seven lysine and arginine residues in PSR-1 PSB. Arrowheads depict three key lysine residues that form a PS-binding interface. *indicates amino acids. (e) Ribbon representation of a modelled PSR-1 structure showing mostly its extracellular domain, in which residues 293–349 are coloured in hot pink. The conserved lysine and arginine residues within PSB are shown as sticks. (g,h) Tryptophan fluorescence quenching assays. The fluorescence quenching titration curves of GST-PSR-1(293–400) with different liposomes containing 10% of the indicated phospholipids (except PC) were determined as described in Methods (g). Briefly, 0.2 μΜ PSR-1 proteins were titrated with different concentrations of liposomes (yaxis) and the fluorescence intensity at 340 nm was plotted against liposomes concentration (see Methods). Liposome models tested were: PC liposomes (67.5% PC, 16% cholesterol, 16.5% sphingomyelin) and PS, PA, PE or PI liposomes (57.5% PC, 16% cholesterol, 16.5% sphingomyelin), in which 10% of the specific phospholipid was included in the liposomes. The fluorescence quenching titration curves of three different PSR-1 proteins with 10% PS liposomes were determined similarly (h). Error bars indicate s.d. (n=3). Figure 1: Identification of a lysine-rich PS-binding motif in PSR-1. ( a ) A schematic cartoon of PSR-1 with its extra- and intracellular domains. The conserved Fe(II)-binding site (H192/D194) and the PS-binding motif (PSB) are shown. ( b , c , f ) In vitro lipid-binding assays. Membrane strips containing equal amounts (500 pmol) of the indicated phospholipids were incubated with 5 μg ml −1 of purified proteins as indicated (see Methods). The lactadherin C2 domain (Lact-C2), known to bind PS, is used as a positive control. After washing three times with washing buffer, the membrane strips were probed with anti-His 6 ( b ) or anti-GST ( c , f ) antibodies. PSR-1 domains and mutations included are as indicated. The strip template on the left depicts phospholipids loaded on the membrane. PS, phosphatidylserine; PC, phosphatidylcholine; PE, phosphatidylethanolamine; PG, phosphatidylglycerol; PA, phosphatidic acid; PI, phosphatidylinositol. ( d ) Sequence alignment of the extracellular domains of PSR proteins from different species. Residues that are identical are indicated in red, residues highly conserved in green, and residues similar in blue. Asterisks indicate seven lysine and arginine residues in PSR-1 PSB. Arrowheads depict three key lysine residues that form a PS-binding interface. *indicates amino acids. ( e ) Ribbon representation of a modelled PSR-1 structure showing mostly its extracellular domain, in which residues 293–349 are coloured in hot pink. The conserved lysine and arginine residues within PSB are shown as sticks. ( g , h ) Tryptophan fluorescence quenching assays. The fluorescence quenching titration curves of GST-PSR-1(293–400) with different liposomes containing 10% of the indicated phospholipids (except PC) were determined as described in Methods ( g ). Briefly, 0.2 μΜ PSR-1 proteins were titrated with different concentrations of liposomes ( y axis) and the fluorescence intensity at 340 nm was plotted against liposomes concentration (see Methods). Liposome models tested were: PC liposomes (67.5% PC, 16% cholesterol, 16.5% sphingomyelin) and PS, PA, PE or PI liposomes (57.5% PC, 16% cholesterol, 16.5% sphingomyelin), in which 10% of the specific phospholipid was included in the liposomes. The fluorescence quenching titration curves of three different PSR-1 proteins with 10% PS liposomes were determined similarly ( h ). Error bars indicate s.d. ( n =3). Full size image We then made deletions in PSR-1(293–400) to define its PS-binding domain and found that GST-PSR-1(293–349) retained the ability to bind PS specifically ( Fig. 1c ). A further deletion from GST-PSR-1(293–349) to GST-PSR-1(293–320) did not seem to affect its PS-binding ability but resulted in reduced binding specificity, as GST-PSR-1(293–320) also showed fairly strong binding to phosphatidic acid (PA; Fig. 1c ). In contrast, GST-PSR-1(321–400) did not bind any phospholipid ( Fig. 1c ). Therefore, residues 293–320 of PSR-1 appear to contain the minimal PS-binding motif. A survey of this 28-residue PS-binding motif, which we call PSB, identifies five lysine residues and two arginine residues (asterisks, Fig. 1d ), which are positively charged and potentially could mediate binding to the negatively charged head group of PS. This PSB motif, and in particular, six of the seven lysine and arginine residues, is highly conserved in PSR proteins across different species ( Fig. 1d ). To gain more insight into the structure of this PSB motif, we modelled C. elegans PSR-1 after the three-dimensional structure of the mouse PSR (also named JMJD6) [33] , [34] . The PSB motif forms a helix-turn-helix (HTH) structure ( Fig. 1e ). Interestingly, three of the five highly conserved lysine residues of PSR-1 (K308, K315 and K319) cluster on one side of the HTH structure, forming a pocket with three positive charges and a potential PS-binding interface ( Fig. 1e ). Two other lysine residues (K305 and K312) and arginine residues (R310 and R320) in PSB appear to scatter on other surfaces of the HTH structure. When two of the three clustered lysine residues were replaced by negatively charged glutamate residues, the resulting mutant protein, GST-PSR-1(293–400; K308E/K315E), failed to bind PS ( Fig. 1c ), indicating that this lysine-rich interface is critical for PS binding. When we mutated the corresponding arginine residues in human PSR (R303 and R310; Fig. 1d ), the resulting human PSR mutant, GST-hPSR(288–403; R303E/R310E), lost its ability to bind PS, compared with the wild-type GST-hPSR(288–403) protein ( Fig. 1f ). This result suggests that the PS-binding motif is conserved in PSR proteins. We confirmed these findings using a tryptophan fluorescence quenching assay. GST-PSR-1(293–400) selectively bound 10% PS liposomes with a dissociation constant ( K d ) of 0.17±0.02 μM ( Fig. 1g and Table 1 ). As expected, K308E/K315E double mutations abolished binding of GST-PSR-1(293–400) to 10% PS liposomes ( Fig. 1h ). Compared with GST-PSR-1(293–400), GST-PSR-1(293-320) bound 10% PS liposomes with a weaker affinity ( K d =0.48±0.17 μM) and lost its lipid-binding specificity ( Fig. 1g and Table 1 ), displaying comparable binding affinity to 10% PA and 10% PE liposomes ( K d =0.59±0.10 μM and 0.40±0.08 μM, respectively). Table 1 Binding affinity ( K d ) of PSR-1 proteins to different liposomes. Full size table PS induces oligomerization of PSR-1 In cell signalling, ligand-induced dimerization or oligomerization of receptors has been a common activation mechanism for cell surface receptors with a single transmembrane domain [35] . We therefore used size-exclusion chromatography to investigate whether PS induces oligomerization of PSR-1, a single transmembrane phagocyte receptor [15] . When GST-PSR-1(293–400) was incubated with 400 μg ml −1 phosphatidylcholine (PC) dissolved in 0.08% mild detergent n -decyl-beta- D -maltopyranoside (DM) or with 0.08% DM alone and then loaded on the Superdex SD200 column, GST-PSR-1(293–400) was eluted in fractions 13–17 ml, which are consistent with the molecular weight of GST-PSR-1(293–400) monomers (arrow, Fig. 2a ). On the other hand, when GST-PSR-1(293–400) was incubated with 400 μg ml −1 PS in 0.08% DM, a significant portion of the protein was found in earlier fractions (fractions 8–12 ml; arrowhead, Fig. 2a ), which indicate significantly larger molecular weights (>232 kDa) and PS-induced oligomerization of GST-PSR-1(293–400). PS-induced oligomerization was not observed with either GST-PSR-1(293–400; K308E/K315E) or GST-PSR-1(321–400; Fig. 2b,c ), which failed to bind PS ( Fig. 1c ), indicating that PS-induced oligomerization of GST-PSR-1(293–400) is dependent on PS-binding. Interestingly, PS induced oligomerization of GST-PSR-1(293–349; arrowhead, Fig. 2e ), which showed a similar PS-binding activity as GST-PSR-1(293–400; Fig. 1c ), but failed to induce oligomerization of GST-PSR-1(293–320), which still bound PS but had a reduced lipid-binding specificity ( Fig. 1c,h and Table 1 ). This result indicates that the adjacent region of PSB (residues 321–349) not only is important for PS-binding specificity, but also is important for PS-induced oligomerization of PSR-1. 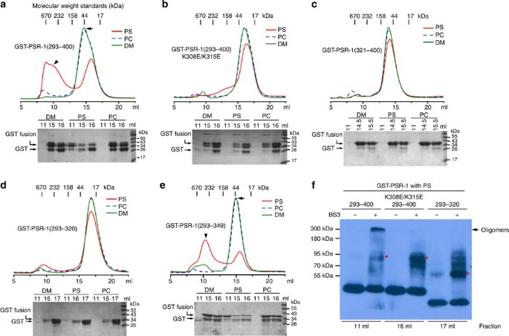Figure 2: PS induces oligomerization of PSR-1. (a–e) PS-induced oligomerization of PSR-1 was analysed by size-exclusion chromatography. Upper panels show the chromatograms of gel filtration. The protein sample (1 mg ml−1) was applied to the Superdex-200 column in a total volume of 1 ml after being incubated with 400 μg ml−1of the indicated phospholipid (dissolved in 0.08% DM) or 0.08% DM alone at 4 °C for 1 h (See Methods). The molecular weight standards indicate the approximate sizes of the proteins in various fractions collected. Three representative fractions were analysed by 15% SDS–PAGE (bottom panels). (f) Crosslinking assays. Chemical crosslinking of the indicated fractions from the size-exclusion chromatography of the indicated GST-PSR-1 proteins incubated with PS was performed as described in Methods. Briefly, protein samples were incubated with or without 25 μM BS3 crosslinker on ice for 60 min and the reactions were terminated and resolved on 8% SDS–PAGE. The arrow indicates the GST-PSR-1(293–400) oligomers. Asterisks indicate potential crosslinked GST-PSR-1 dimers, as GST fusion proteins are known to form homodimers in solution62. Figure 2: PS induces oligomerization of PSR-1. ( a – e ) PS-induced oligomerization of PSR-1 was analysed by size-exclusion chromatography. Upper panels show the chromatograms of gel filtration. The protein sample (1 mg ml −1 ) was applied to the Superdex-200 column in a total volume of 1 ml after being incubated with 400 μg ml −1 of the indicated phospholipid (dissolved in 0.08% DM) or 0.08% DM alone at 4 °C for 1 h (See Methods). The molecular weight standards indicate the approximate sizes of the proteins in various fractions collected. Three representative fractions were analysed by 15% SDS–PAGE (bottom panels). ( f ) Crosslinking assays. Chemical crosslinking of the indicated fractions from the size-exclusion chromatography of the indicated GST-PSR-1 proteins incubated with PS was performed as described in Methods. Briefly, protein samples were incubated with or without 25 μM BS3 crosslinker on ice for 60 min and the reactions were terminated and resolved on 8% SDS–PAGE. The arrow indicates the GST-PSR-1(293–400) oligomers. Asterisks indicate potential crosslinked GST-PSR-1 dimers, as GST fusion proteins are known to form homodimers in solution [62] . Full size image We confirmed these findings using chemical crosslinking experiments. When the 11 ml fraction of GST-PSR-1(293–400) with PS was treated with an amine-reactive crosslinker Bis[sulfosuccinimidyl] suberate (BS3), a major crosslinked band at ~300 kDa was observed ( Fig. 2f ), which is consistent with the estimated size of GST-PSR-1(293–400) oligomers from size-exclusion chromatography ( Fig. 2a ). In contrast, no oligomer formation was observed with either GST-PSR-1(293–400; K308E/K315E) or GST-PSR-1(293–320), when their monomer fractions (16 and 17 ml fractions, respectively) were treated with BS3 ( Fig. 2f ), indicating that GST-PSR-1(293–400; K308E/K315E) or GST-PSR-1(293–320) does not undergo PS-induced oligomerization. PSR-1 is important for clearance of apoptotic germ cells We next examined the importance of the PSB motif to the function of PSR-1 in C. elegans . Previous studies have shown that PSR-1 promotes phagocytosis of somatic apoptotic cells by recognizing PS exposed on the surface of apoptotic cells and transducing the ‘eat-me’ signal through direct interaction with two downstream signalling components, CED-5 and CED-12 (ref. 23 ). However, the engulfment defect caused by the strong loss-of-function ( lf ) psr-1(tm469) mutation is weak, probably due to the presence of other ‘eat-me’ signals and additional phagocyte receptors acting in parallel [1] , [36] , which could significantly reduce the impact of psr-1 inactivation to clearance of apoptotic cells. Indeed, when PS is the only signal exposed on the surface of living cells in animals deficient in tat-1, which encodes a P-type ATPase critical for maintaining plasma membrane PS asymmetry, psr-1(tm469) completely blocks phagocytic removal of PS-exposed living cells by neighbouring cells [24] . We examined the role of psr-1 in promoting engulfment of apoptotic cells in C. elegans germ line, which shares key activators and effectors of apoptosis with the soma [37] . Although psr-1(tm469) alone did not seem to affect clearance of apoptotic germ cells, it mildly increased the number of germ cell corpses after ultraviolet irradiation compared with that seen in wild-type animals irradiated with ultraviolet ( Supplementary Fig. 1 ). Strikingly, psr-1(tm469) markedly increased the number of unengulfed germ cell corpses in strong lf mutants defective in the ced-1, ced-6 or ced-7 gene ( Fig. 3a–c ), all of which act in the same pathway to promote clearance of apoptotic cells [38] , indicating that psr-1 does not act in the ced-1, ced-6 and ced-7 engulfment pathway. In comparison, psr-1(tm469) did not alter the number of unengulfed germ cell corpses in strong lf mutants deficient in the ced-2, ced-5 or ced-12 genes ( Fig. 3d–f ), which act in an engulfment pathway parallel to the CED-1 pathway [38] . These results confirm the finding from analysis in somatic cells that psr-1 acts in the ced-2, ced-5 and ced-12 pathway to promote phagocytosis of apoptotic cells [23] . Time-lapse microscopy analysis of the durations of germ cell corpses in wild-type and psr-1(tm469) animals reveals that on average germ cell corpses in wild-type N2 animals persisted for 30 min, ranging from 16 to 42 min. In contrast, germ cell corpses in psr-1(tm469) animals lasted for an average of 60 min (ranging from 35 to 130 min), which is twice as long as that of N2 animals ( Fig. 3g ). This result further indicates that the loss of psr-1 compromises clearance of germ cell corpses. It is interesting that psr-1(tm469) markedly enhances the engulfment defect of the ced-1, ced-6 and ced-7 pathway in the germ line, but only mildly enhances the engulfment defect of the ced-1, ced-6 and ced-7 pathway in the soma [23] . In fact, the number of persistent germ cell corpses in the ced-1(e1735) ; psr-1(tm469) double mutant is almost identical to that observed in ced-1(e1735) ; ced-2(e1752) double mutant ( Fig. 3h ), which is defective in both engulfment pathways. This surprising result indicates that loss of psr-1 in the ced-1(e1735) mutant background has as big an impact to clearance of germ cell corpses as loss of the entire ced-2 engulfment pathway. It is possible that a component acting in parallel to psr-1 in the soma does not function in the germ line, which then exacerbates the engulfment defect caused by simultaneous loss of psr-1 and the ced-1 pathway in the germline. 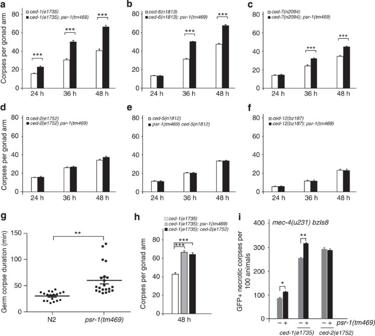Figure 3:psr-1promotes the clearance of necrotic and apoptotic germ cells through the CED-2 pathway. (a–f,h) Time-course analysis of germ cell corpses duringC. elegansgermline development. Germ cell corpses from the indicated strains were scored at 24, 36 and 48 h post L4 to the adult molt from one gonad arm of the animals. Theyaxis represents the mean number of cell corpses scored at the time point indicated on thexaxis. Error bars indicate s.e.m (n=15 at each time point). (g) Time-lapse microscopy analysis of durations of persistent germ cell corpses. The persistence of germ cell corpses from wild-type N2 animals (20 corpses) andpsr-1(tm469)animals (21 corpses) was monitored. Theyaxis indicates the persistence time for each germ cell corpse. The mean persistence time of germ cell corpses for each genotype was also shown. Error bars indicate s.e.m. The numbers of eggs laid by N2 andpsr-1(tm469)animals at 24, 36 and 48 h post L4 to the adult molt were counted to ensure that the germlines of the two strains had similar rates of development (Supplementary Fig. 2). (i)psr-1acts in theced-2pathway to promote clearance of necrotic cell corpses. The numbers of GFP-positive, unengulfed necrotic cell corpses with vacuolar morphology in the indicated strains were scored in L4 larvae. All strains containmec-4(u231) bzIs8.Theyaxis represents the mean number from three independent experiments for each genotype. Error bars indicate s.e.m (n=100 each strain). In all panels, the significance of differences between results was determined by Student’st-tests, *P<0.01; **P<0.001; ***P<0.0001. Figure 3: psr-1 promotes the clearance of necrotic and apoptotic germ cells through the CED-2 pathway. ( a – f , h ) Time-course analysis of germ cell corpses during C. elegans germline development. Germ cell corpses from the indicated strains were scored at 24, 36 and 48 h post L4 to the adult molt from one gonad arm of the animals. The y axis represents the mean number of cell corpses scored at the time point indicated on the x axis. Error bars indicate s.e.m ( n =15 at each time point). ( g ) Time-lapse microscopy analysis of durations of persistent germ cell corpses. The persistence of germ cell corpses from wild-type N2 animals (20 corpses) and psr-1(tm469) animals (21 corpses) was monitored. The y axis indicates the persistence time for each germ cell corpse. The mean persistence time of germ cell corpses for each genotype was also shown. Error bars indicate s.e.m. The numbers of eggs laid by N2 and psr-1(tm469) animals at 24, 36 and 48 h post L4 to the adult molt were counted to ensure that the germlines of the two strains had similar rates of development ( Supplementary Fig. 2 ). ( i ) psr-1 acts in the ced-2 pathway to promote clearance of necrotic cell corpses. The numbers of GFP-positive, unengulfed necrotic cell corpses with vacuolar morphology in the indicated strains were scored in L4 larvae. All strains contain mec-4(u231) bzIs8. The y axis represents the mean number from three independent experiments for each genotype. Error bars indicate s.e.m ( n =100 each strain). In all panels, the significance of differences between results was determined by Student’s t -tests, * P <0.01; ** P <0.001; *** P <0.0001. Full size image PSR-1 is important for clearance of necrotic cell corpses The two parallel-acting phagocytosis pathways not only are responsible for clearing apoptotic cells during development, but also contribute to the clearance of necrotic cell corpses [39] . We thus investigated whether psr-1 also affects clearance of necrotic cells. A gain-of-function mutation (u231) in the mec-4 gene causes necrotic death of six mechanosensory neurons, which can be labelled and tracked by an integrated transgene bzIs8 that expresses green fluorescent protein (GFP) in these six neurons under the control of the mec-4 gene promoter (P mec-4 GFP) [39] ( Supplementary Fig. 3 ). We quantified the number of GFP-positive, vacuolar necrotic corpses in mec-4(u231) bzIs8 larvae or mec-4(u231) bzIs8 larvae that are also deficient in psr-1 , ced-1, or ced-2 , or doubly deficient in psr-1 and ced-1 or psr-1 and ced-2 . Consistent with the previous report [39] , loss of either ced-1 or ced-2 greatly delayed the removal of GFP-positive necrotic corpses ( Fig. 3i ). In comparison, loss of psr-1 caused a mild but significant delay in clearance of necrotic corpses. psr-1(tm469) markedly enhanced the persistence of necrotic corpses caused by loss of ced-1 but not that caused by loss of ced-2 ( Fig. 3i ). Therefore, as in somatic and germ cell death, psr-1 acts in the ced-2 phagocytosis pathway to promote clearance of necrotic cells. The PS-binding motif of PSR-1 is required for cell clearance Because mammalian PSR has been shown to act as a histone arginine demethylase, a lysyl hydroxylase, or a ssRNA-binding protein [31] , [32] , [33] , we examined whether these different PSR activities and the PS-binding motif of PSR-1 are important for clearance of apoptotic cells in C. elegans . To rule out the concern of transgene overexpression, we generated transgenic animals carrying a single-copy insertion (SCI) of a 9.4-kb psr-1 genomic fragment, which contains 2,321 bp psr-1 coding region, 1,972 bp 3′ untranslated region of psr-1 , two upstream genes ( ubc-9 and F29B9.5) in the polycistronic operon and 2,777 bp promoter upstream of the operon. We generated psr-1 SCIs inserted at the same chromosomal location, which contained either the K308E/K315E substitutions in the PSB motif or the H192A/D194A mutations in the JmjC domain that alter two highly conserved residues required for Fe(II) binding and the demethylase or the hydroxylase activity of PSR [31] , [32] . When introduced into the ced-1(e1735); psr-1(tm469) mutant, the wild-type psr-1 SCI alleviated the severe defect of germ cell corpse clearance in the double mutant to the level seen in the ced-1(e1735) single mutant ( Fig. 4a ), indicating full rescue of the engulfment defect contributed by psr-1(tm469) . The psr-1 SCI carrying the H192A/D194A substitutions also fully rescued the engulfment defect contributed by psr-1(tm469) in the double mutant ( Fig. 4a ), indicating that the Fe(II)-dependent biochemical activity of PSR-1 is dispensable for the cell corpse clearance function of PSR-1. In contrast, the psr-1 SCI harbouring the K308E/K315E substitutions in the PSB motif failed to rescue the engulfment defect contributed by psr-1(tm469) ( Fig. 4a ), indicating that the PSB motif is critical for the cell corpse engulfment function of PSR-1. 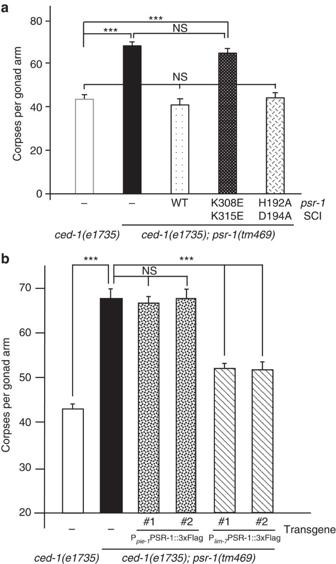Figure 4: The PS-binding motif of PSR-1 is required for the clearance of apoptotic cells. (a,b) The number of germ cell corpses per gonad arm was scored in the indicated strains at 48 h post L4 to the adult molt as described inFig. 3. SCI indicates single copy insertion of thepsr-1transgene (a). Complex transgenic arrays containing Ppie-1PSR-1::3xFlag, which directs PSR-1::3xFlag expression in germ cells under the control of the germline-specificpie-1promoter9, and transgenic arrays harbouring Plim-7PSR-1::3xFlag, which directs PSR-1::3xFlag expression in gonadal sheath cells under the control of thelim-7promoter42, were used to assist determination of the PSR-1 acting site (b). Theyaxis represents the average number of germ cell corpses. Error bars are s.e.m (n=15 each strain). Two independent transgenic lines were analysed (b). The significance of differences between results was determined by Student’st-tests, ***P<0.0001. NS indicates no significant difference. Figure 4: The PS-binding motif of PSR-1 is required for the clearance of apoptotic cells. ( a , b ) The number of germ cell corpses per gonad arm was scored in the indicated strains at 48 h post L4 to the adult molt as described in Fig. 3 . SCI indicates single copy insertion of the psr-1 transgene ( a ). Complex transgenic arrays containing P pie-1 PSR-1::3xFlag, which directs PSR-1::3xFlag expression in germ cells under the control of the germline-specific pie-1 promoter [9] , and transgenic arrays harbouring P lim-7 PSR-1::3xFlag, which directs PSR-1::3xFlag expression in gonadal sheath cells under the control of the lim-7 promoter [42] , were used to assist determination of the PSR-1 acting site ( b ). The y axis represents the average number of germ cell corpses. Error bars are s.e.m ( n =15 each strain). Two independent transgenic lines were analysed ( b ). The significance of differences between results was determined by Student’s t -tests, *** P <0.0001. NS indicates no significant difference. Full size image To ascertain that the above mutations in the psr-1 gene did not alter the expression level or the stability of the PSR-1 protein, we raised 13 mouse monoclonal antibodies and eight rat polyclonal antibodies against PSR-1 ( Supplementary Fig. 4a–c ). All of them detected recombinant PSR-1 proteins with high affinity ( Supplementary Fig. 4a–c ), but failed to detect the endogenous PSR-1 protein in worm lysates by immunoblotting ( Supplementary Fig. 4b,c ) or in animals by immunostaining ( Supplementary Fig. 5a ). The inability to detect endogenous PSR-1 using these 21 antibodies suggests that in vivo PSR-1 either is expressed at a very low level or is unstable or both. Real-time reverse transcription-PCR analysis of psr-1 transcripts indicates that the mRNA level of psr-1 is ~1/4 of that of the ced-1 gene and 1/100 of that of the housekeeping gene rpl-26 ( Supplementary Fig. 4d ). We then generated several psr-1 SCIs with a 3xFlag epitope, which allows the detection of the femtomole level of the tagged protein by immunoblotting [40] , attached to the N terminus of PSR-1. As shown in Supplementary Fig. 4e , a monoclonal M2 antibody to the Flag epitope detected a protein slightly larger than 50 kDa in 3xflag::psr-1 SCI animals, which was close to the predicted size of 3xFlag::PSR-1 and was absent in N2 animals. One additional band of a lower molecular weight was observed in both 3xflag::psr-1 SCI animals and N2 animals, indicating that it is a protein cross-reacting to the M2 antibody and not related to PSR-1. In 3xflag::psr-1 SCI animals carrying K308E/K315E substitutions or H192A/D194A substitutions, the PSR-1 protein levels were comparable to that in wild-type 3xflag::psr-1 SCI animals ( Supplementary Fig. 4e ), indicating that these mutations do not affect the expression level or the stability of PSR-1. Taken together, these results indicate that the PS-binding activity of PSR-1, but not its Fe(II)-dependent biochemical activities, is required for PSR-1 to promote cell corpse clearance. PSR-1 enriches on and clusters around apoptotic cells We next examined the subcellular localization and the membrane topology of PSR-1, a predicted type II transmembrane protein [15] using the 3xflag::psr-1 SCI and a psr-1::3xflag SCI, in which the 3xFlag epitope is fused to the C terminus of PSR-1. The expression levels of PSR-1 from these two psr-1 SCI transgenes were similar ( Supplementary Fig. 4f ). Because psr-1 plays a more prominent role in clearance of germ cell corpses, we first examined where PSR-1 acts to mediate clearance of apoptotic germ cells. Expression of PSR-1::3xFlag in germ cells under the control of the germline-specific pie-1 promoter failed to rescue the engulfment defect contributed by psr-1(tm469) in the ced-1(e1735); psr-1(tm469) double mutant, whereas the expression of PSR-1::3xFlag in gonadal sheath cells, which serve as phagocytes to remove apoptotic germ cells [37] , [41] , under the control of the lim-7 promoter could rescue [42] ( Fig. 4b ). These results indicate that PSR-1 acts in gonadal sheath cells to promote clearance of germ cell corpses. In 3xflag::psr-1 SCI, psr-1::3xflag SCI, or N2 animals, we did not detect any specific staining in germ cells or tightly attached gonadal sheath cells using the Anti-Flag M2 antibody ( Supplementary Fig. 5b ). Neither did we observe any specific staining in embryos from 3xflag::psr-1 SCI, psr-1::3xflag SCI or N2 animals ( Supplementary Fig. 5c ). These results are consistent with the observations that the PSR-1 protein is present at a very low level in animals and are very difficult to detect ( Supplementary Fig. 4a–d ). Because phagocyte receptors often enrich on the surface of phagocytes in contact with apoptotic cells and cluster around apoptotic cells [36] , [43] , we performed immunostaining on dissected C. elegans gonads with persistent germ cell corpses using non-permeabilized conditions, which allow examination of the membrane topology of PSR-1. As expected, we did not see any specific staining using the anti-Flag M2 antibody in dissected gonads from ced-1(e1735) ; psr-1(tm469) animals ( Fig. 5a ), which did not carry any Flag-tagged psr-1 SCI. On the other hand, we consistently observed M2 staining in clusters on the surface of 4 to 11 apoptotic germ cells in dissected gonads from ced-1(e1735) ; psr-1::3xflag SCI; psr-1(tm469) animals ( Fig. 5c ). These PSR-1::3xFlag staining puncta resembled those of the CED-1 phagocyte receptor tagged with GFP (CED-1ΔC::GFP) and co-localized with CED-1ΔC::GFP on the surface of apoptotic cells ( Supplementary Fig. 5d ), confirming that PSR-1 selectively clusters on the surface of apoptotic cells. In contrast, we did not observe any M2 staining in dissected gonads from ced-1(e1735); 3xflag::psr-1 SCI; psr-1(tm469) animals ( Fig. 5b ), which carried a different psr-1 SCI with an N-terminal 3xFlag tag. These results confirm the predicted membrane topology of PSR-1, which has its C terminus in the extracellular space, accessible to M2 antibody staining, and its N terminus in the cytoplasm, which is not accessible to the antibody in non-permeabilized conditions. The low number of apoptotic cells stained by the M2 antibody in dissected gonads from ced-1(e1735) ; psr-1::3xflag SCI; psr-1(tm469) animals is probably due to the very low expression level of PSR-1, which normally could not be detected, but became concentrated on the surface of some phagocytes that surrounded the apoptotic cells. Moreover, the clustering of phagocyte receptors on apoptotic cells could be transient, as human PSR also transiently appears on the surface of the THP-1 phagocytes after phorbol 12-myristate 13 acetate activation, and this cell surface PSR expression is important for engulfment of dead cell corpses by THP-1 phagocytes [20] . 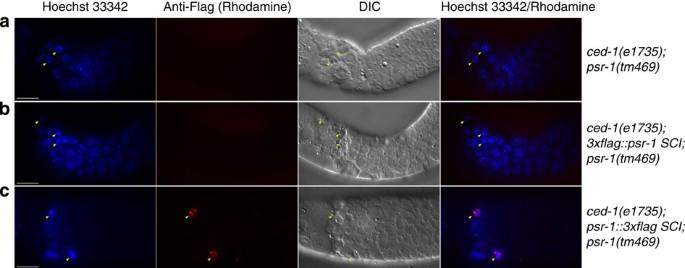Figure 5: PSR-1 enriches and clusters on the surface of apoptotic germ cells. (a–c) Adult hermaphrodites of the indicated genotypes (24 h post L4 to the adult molt) were dissected to expose their gonads, which were then stained with Hoechst 33342 and an anti-Flag M2 antibody using non-permeabilized conditions (see Methods). Images of Hoechst 33342, anti-Flag (Rhodamine), DIC and the merged image of Rhodamine/Hoechst are shown. Arrowheads indicate apoptotic germ cells with characteristic condensed Hoechst staining and distinct corpse morphology under DIC. Scale bars, 10 μm. Figure 5: PSR-1 enriches and clusters on the surface of apoptotic germ cells. ( a – c ) Adult hermaphrodites of the indicated genotypes (24 h post L4 to the adult molt) were dissected to expose their gonads, which were then stained with Hoechst 33342 and an anti-Flag M2 antibody using non-permeabilized conditions (see Methods). Images of Hoechst 33342, anti-Flag (Rhodamine), DIC and the merged image of Rhodamine/Hoechst are shown. Arrowheads indicate apoptotic germ cells with characteristic condensed Hoechst staining and distinct corpse morphology under DIC. Scale bars, 10 μm. Full size image We also took advantage of the 3xflag::psr-1 SCI animals to examine if PSR-1 acts in the CED-2, CED-5 and CED-12 engulfment pathway by recruiting the CED-2, CED-5 and CED-12 ternary signalling complex [23] , [44] , [45] , [46] . Co-immunoprecipitation was performed in 3xflag::psr-1 SCI animals and animals carrying an integrated transgene ( smIs350 ) expressing TRA-2::3xFlag, a single transmembrane receptor important for C. elegans sex determination [47] . The M2 antibody specifically co-precipitated the endogenous CED-2 protein with 3xFlag::PSR-1, but not with TRA-2::3xFlag ( Supplementary Fig. 6 ). This result provides further support that PSR-1 acts through the CED-2, CED-5 and CED-12 pathway to promote clearance of dead cells. To date, PSR has been reported to function as a PS-recognizing phagocyte receptor, a histone arginine demethylase, a lysyl hydroxylase or a ssRNA-binding protein [15] , [23] , [31] , [32] , [33] . Although there are extensive debates on some of these proposed activities or functions and the in vivo significance of these activities [16] , [18] , [25] , [26] , [27] , [31] , [32] , [33] , it is generally accepted that PSR is a conserved and multifunctional protein that plays important roles in animal development and tissue homeostasis. In this study, we provide new and strong evidence that C. elegans PSR-1 acts in the ced-2, ced-5 and ced-12 signalling pathway to promote clearance of apoptotic germ cells and necrotic cells, in addition to its role in clearance of somatic apoptotic cells. More importantly, we identify a conserved and previously uncharacterized PS-binding motif in the extracellular domain of PSR-1 that is critical for its function in clearance of apoptotic cells. Although in mammals several other membrane proteins, including BAI1, TIM4 and stabilin-2 (refs 28 , 29 , 30 ), have been proposed to be potential PS receptors, none of these mammalian proteins, except PSR, has a corresponding homologue in C. elegans , indicating that they are not the conserved PS receptor central to apoptotic corpse clearance in diverse organisms [14] . Therefore, our study suggests that PSR is the best candidate for the conserved PS receptor. The subcellular localization pattern of PSR is a subject of great interest because it is closely related to the physiological functions of PSR. Human PSR has been reported to localize to the plasma membrane, nuclei or both [15] , [20] , [48] . In C. elegans , the PSR-1 protein appears to be present at an extremely low level, as it cannot be detected by more than 20 different monoclonal and polyclonal antibodies raised against PSR-1 that show high affinity to recombinant PSR-1 ( Supplementary Fig. 4a–c and Fig. 5a ). Using a single-copy psr-1 transgene tagged with an ultrasensitive 3xFlag epitope, we were able to detect PSR-1 expression in C. elegans by immunoblotting ( Supplementary Fig. 4e,f ), but failed to see PSR-1 in living cells by immunostaining ( Fig. 5 and Supplementary Fig. 5b,c ). Importantly, we did observe that PSR-1 concentrated on the surface of some apoptotic germ cells and formed a punctate circle on apoptotic cells, similar to that formed by the CED-1 phagocyte receptor ( Fig. 5 and Supplementary Fig. 5d ) [43] . These observations are consistent with PSR-1 serving as a phagocyte receptor that oligomerizes and aggregates upon binding to exposed PS on the surface of apoptotic cells ( Fig. 2 ) and triggers phagocytosis by recruiting the CED-2/CED-5/CED-12 ternary signalling complex ( Supplementary Fig. 6 ). Moreover, using non-permeabilized staining conditions and two different single-copy psr-1 transgenes, in which PSR-1 is tagged at its N terminus and C terminus with the 3xFlag epitope, respectively, we confirm the predicted membrane topology of PSR-1, with its N-terminal portion in the cytosol and its C-terminal portion in the extracellular space. Taken together, these results establish that PSR-1 is a PS-recognizing membrane receptor important for phagocytosis of apoptotic cells. As expected, the PS-binding motif in the extracellular domain of PSR-1 is required for its cell corpse clearance function. Intriguingly, the Fe(II)-binding site in the intracellular domain of PSR-1, critical for the JmjC activities, is dispensable for its phagocytosis function. This result suggests that the Fe(II)-dependent demethylase or hydroxylase activity of PSR is not involved in cell corpse clearance and is in line with the finding that the intracellular domain of PSR-1 directly interacts with CED-5 and CED-12 in the ced-2, ced-5 and ced-12 phagocytosis pathway, which form a ternary complex in response to upstream phagocytosis signals to activate cytoskeletal rearrangement and membrane extension required for phagocytosis ( Fig. 6 ) [44] , [46] , [49] . Perhaps, PS-induced oligomerization of PSR-1 is sufficient to trigger this signalling cascade. Interestingly, PSR-1 is also critical for axonal fusion during regeneration of neurons with severed axons [50] , which requires the PS-binding motif of PSR-1 to recognize the PS ‘save-me’ signal exposed on the surface of the severed distal axon fragment as well as the Fe(II)-dependent activities of PSR-1 that are dispensable for clearance of apoptotic cells. Therefore, C. elegans PSR-1 functions in both apoptotic and non-apoptotic processes to regulate animal development and tissue homeostasis, through a shared PS-mediated mechanism. 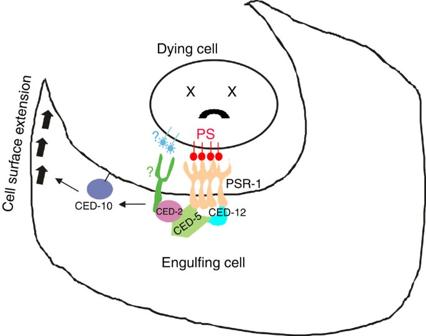Figure 6: Model of PSR-1-mediated clearance of apoptotic cells. PS exposed on the surface of the apoptotic cell interacts with and induces the oligomerization of PSR-1, which then transduces the ‘eat-me’ signal through interacting with CED-5 and CED-12, leading to the activation of the CED-10 GTPase and membrane extension of the phagocyte to enclose and internalize the apoptotic cell. At least one unknown phagocyte receptor (?) acts in parallel to PSR-1 in this signalling pathway. Figure 6: Model of PSR-1-mediated clearance of apoptotic cells. PS exposed on the surface of the apoptotic cell interacts with and induces the oligomerization of PSR-1, which then transduces the ‘eat-me’ signal through interacting with CED-5 and CED-12, leading to the activation of the CED-10 GTPase and membrane extension of the phagocyte to enclose and internalize the apoptotic cell. At least one unknown phagocyte receptor (?) acts in parallel to PSR-1 in this signalling pathway. Full size image Strains C. elegans strains were maintained using standard methods [51] . All alleles used for this study have been described in detail [52] , except for those SCI psr-1 transgenes, which were all inserted at the same position on Linkage Group II (ref. 53 ). These are smIs488 (wild-type psr-1 ), smIs491 ( psr-1 with H192A/D194A), smIs492 (psr-1 with K308E/K315E), smIs490 (psr-1::3xflag) , smIs510 (3xflag::psr-1) , smIs511(3xflag::psr-1) , smIs513(3xflag::psr-1 with H192A/D194A) and smIs514(3xflag::psr-1 with K308E/K315E). Detailed information on smIs350 (LGIV) and bzIs8 (LGX) have been reported [24] , [54] . Quantification of necrotic and germ cell corpses The number of germ cell corpses in one gonad arm from animals at various adult ages was scored using Nomarski optics [41] . L4 mutant larvae carrying mec-4(u231) bzIs8 were examined for the presence of GFP-labelled cell corpses using a fluorescent Nomarski microscope to quantify the number of persistent necrotic cell corpses. For cell corpse assays, we normally scored 15 animals at each time point for germ cell corpses or 100 L4 larvae for necrotic cell corpses in each strain, which are sufficient to allow us to detect minor difference in cell death. Quantification of ultraviolet irradiation-induced germ cell corpses To assess the effects of ultraviolet on germ cell apoptosis, worms were allowed to develop to the young adult stage (24 h after L4 to the adult molt) at 20 °C, treated with 100 Jm −2 ultraviolet on non-seeded NGM plates using a Stratalinker (Stratagene, Inc.). Immediately after ultraviolet irradiation, worms were transferred to fresh NGM plates and germ cell corpses were scored by Nomarski optic in the pachytene region of the gonads 2, 4 or 6 h later. Transgenic animals The P lim-7 PSR-1::3xFlag construct (at 25 ng μl −1 ) was injected into ced-1(e1735); psr-1(tm469) animals, using P sur-5 GFP (25 ng μl −1 ) and pRF4 (25 ng μl −1 ) as transgenic markers. The P pie-1 PSR-1::3xFlag construct (at 5 ng μl −1 ) was injected into the ced-1(e1735); psr-1(tm469) animals using a complex genomic array method, which allows the germ line expression of transgene [9] , using P sur-5 GFP (25 ng μl −1 ) and pRF4 (25 ng μl −1 ) as a transgenic marker. The P ced-1 CED-1ΔC::GFP construct (at 25 ng μl −1 ) was injected into ced-1(e1735) ; smIs490 ; psr-1(tm469) animals using pRF4 (25 ng μl −1 ) as a transgenic marker. Time lapse microscopy Adult animals 24 h post the L4 to adult molt were mounted on slides with agar pads in S-Basal (100 mM NaCl, 7.3 mM K 2 HPO 4 , 34 mM KH 2 PO 4 , 5 mg l −1 cholesterol) with 5 mM Levamisole. Cover slips were sealed with Beeswax and Vaseline (1:1). Images in a z series of 1 μm per layer were captured every minute for 3 h using a Zeiss Axioplan 2 microscope equipped with a Cohu CCD camera and a Slidebook 5 software. Structural modelling of PSR-1 The three-dimensional model of full-length C. elegans PSR-1 was constructed based on the determined structure of mammalian PSR using the comparative modelling tool Modeler 9.9 (refs 33 , 34 , 55 ). The public online server I-TASSER was also used to obtain more predictions [56] . The top predicted models derived from Modeler and I-TASSER were minimized using the simulation package GROMACS 4.5 (ref. 57 ), and the final model with lower energy after minimization was selected as the PSR-1 modelled structure. The structure figure was generated by the PyMOL programme ( http://www.pymol.org ). Molecular biology Standard methods of cloning, sequencing and PCR amplification were used. A 9,411-bp psr-1 operon was excised from fosmid WRM0629aB05 through SpeI and AgeI digestion and subcloned into the pSL1190 vector through the same restriction sites to make the construct pSL1190- psr-1 . Mutations or the 3xFlag epitope were generated in this construct through in vitro mutagenesis and the constructs were confirmed by DNA sequencing. The 9,411-bp wild-type or altered psr-1 fragment was then subcloned into the pCFJ151 vector to generate template constructs for Mos transposase-mediated SCI [53] . The psr-1::3xflag coding region was PCR amplified using primers 5′-ATGGATTCATGTCATTAGGGCGAGATAG-3′ and 5′-ATACTAGGGGCCCTTTCAAATTCGAACAAGTTTAATTCGTG-3′ and the psr-1::3xflag SCI construct as the template. This psr-1::3xflag PCR fragment was then inserted into the pTE5 vector (P pie-1 GFP) through its SpeI and ApaI sites to generate the P pie-1 PSR-1::3xFlag construct and a pPD49.26 vector containing the lim-7 promoter and intron 1 through its BamHI and SpeI sites to generate the P lim-7 PSR-1::3xFlag construct. RNA extraction and real-time PCR analysis of mRNA levels C. elegans animals were washed off plates with M9 buffer and collected in 15 ml conical tubes. After centrifugation, the worm pellets were washed three times with M9 buffer to remove bacteria. Trizol (Takara Bio) was added to the worm pellets, which after vortexing were placed in liquid nitrogen and thawed at 37 °C for six times. After that, total RNA was extracted following the instructions of the manufacturer (Takara Bio). Total RNA (2 μg) was used for cDNA synthesis using the Oligo-d(T) 15 primer. Real-time PCR analysis was performed on the rpl-26 , ced-1 and psr-1 genes using the CFX96 Real-Time PCR Detection System (Bio-Rad) and iTaq Universal SYBR Green Supermix reagents (Bio-Rad). PCR reactions were run in triplicate and three independent experiments were performed. The mean mRNA level of the housekeeping gene rpl-26 was used as a control to normalize the variability in expression levels. Primer sequences used in real-time PCR reactions were: rpl-26 forward primer 5′-ATGAAGGTCAAT-CCGTTCGT-3′ and reverse primer 5′-AGGACACGTCCAGTGTTTCC-3′; ced-1 forward primer 5′-CTGCAATTGGCTGCTGCCATGTAGA-3′ and reverse primer 5′-AGACCATTGGGTGGTCCTCCTTGAT-3′; and psr-1 forward primer 5′-CATGC-GAAGGACAAAGCGAG-3′ and reverse primer 5′-CGAAATCTCGGCGGAACTCC-3′. Generation of SCI In brief, young adult EG4322 animals ( ttTi5605 ; unc-119 ( ed9 )) were injected with 25 ng μl −1 of the wild-type or altered pCFJ151- psr-1 construct, 25 ng μl −1 pJL43.1 (P glh-2 transposase), 5 ng μl −1 pCFJ70 [ Pmyo-3 twk-18(cn110)], 5 ng μl −1 of pCFJ104 (P myo-3 mCherry) and 5 ng μl −1 of pCFJ90 (P myo-2 mCherry). F1 non-Unc animals were cloned out and cultured at 16 °C. After two generations, the animals were shifted to 25 °C for 1–2 days. The non-Unc animals without any Cherry expression were selected as candidate SCI lines, which were first examined by PCR using the following primer set: SCIs, 5′-TCTGGCTCTGCTTCTTCGTT-3′ and SCIas: 5′-CAATTCATCCCGGTTTCTGT-3′. Those lines that produced 1.8 kb PCR products indicate occurring of recombination between the chromosome and the plasmid templates and were further examined for SCI through long-range PCR (Takara’s LA PCR Kit, Clontech) for the expected length of insertion using the primer set: SCIs and SCIas2: 5′-GAACCTAACTGTAAAAGTCCAC-3′. Some of the SCI lines were further confirmed by quantitative PCR using a Rotor-gene 3000 machine (Corbett, Australia) and SYBR Green JumpStart (Sigma, St Louis, MO). The genomic DNA from homozygous transgenic animals was extracted and used as templates. Two primer sets, one from the nuc-1 gene (used as an internal control) and one from the psr-1 gene, were used to quantify the copy number of the insertion. The primer sequences are: nuc-1 qPCRs: 5′-GGAACTTCTGGAGTCTGGTTGG-3′, nuc-1 qPCRas: 5′-GTCCTTT-TTGGTATTGTCCAGCG-3′, psr-1 qPCRs: 5′-CGGCACGGAAAAGTGGACGTGG-3′, psr-1 qPCRas: 5′-GACTCGTTCATATCATAGAGCGGG-3′. Generation of mouse monoclonal antibodies to PSR-1 In brief, monoclonal antibodies to PSR-1 were raised in mice using a subcutaneous injection of 100 μg of the purified GST-PSR-1(293–400) protein emulsified in Freund’s complete adjuvant, which is followed by an intravenous booster injection of 50 μg GST-PSR-1(293–400) 2 weeks later. The resulting hybridomas were screened for the secretion of monoclonal antibodies specific to GST-PSR-1(293–400) using an indirect enzyme-linked immunosorbent assay. Positive clones were expanded and cultured in 75-cm 2 flasks. Cells producing monoclonal antibodies were then cloned by limiting dilution at least three times. Monoclonal antibodies were prepared by injecting hybridoma cultures into the peritoneal cavities of pristine-primed BALB/c mice; ascites were collected after 9–12 days and stored at −20 °C. Monoclonal antibodies were purified from the collected ascites using ammonium sulfate precipitation followed by Mabselect-Xtral affinity chromatography (Amersham GE Health, Uppsala, Sweden). Immunoglobulin concentrations were determined on a DU800 spectrophotometer (Beckman Coulters, California, USA). Western blot analysis 100 L4 larvae from each strain were transferred into 30 μl of 2 × SDS–polyacrylamide gel electrophoresis (PAGE) loading buffer, subjected to the freeze-thaw treatment three times in liquid nitrogen and water bath and then incubated in 65 °C for 30 min. The samples were resolved on 12% SDS–PAGE, transferred to a polyvinylidene fluoride (PVDF) membrane and subjected to the western blot analysis using anti-Flag M2 monoclonal antibody (Sigma-Aldrich, Cat. No. F3165; 1:5,000 dilution). The blotted membrane was then treated with a stripping buffer (50 mM Tris-HCl, pH6.8, 2% SDS and 200 mM DTT) at 65 °C for 30 min to remove the M2 antibody and reprobed with anti-tubulin monoclonal antibody (Developmental Studies Hybridoma Bank, Cat. No. 12G10; 1:3000 dilution) to examine the expression levels of alpha-tubulin as a loading control. Uncropped scans of all western blots are provided in Supplementary Fig. 7 . The enzyme-linked immunosorbent assay (ELISA) To evaluate the reactivity and specificity of monoclonal antibodies to PSR-1, 0.2 μg per well of recombinant GST-PSR-1(293–400) or GST were coated on polystyrene plates. Antibodies were diluted to 0.1 μg ml −1 and then analysed by indirect ELISA following the standard protocols [58] . Immunostaining For non-permeabilized staining, gonads of hermaphrodites were gently dissected out by cutting the hermaphrodites at the head in a depression slide while immersed in the staining buffer (PBS containing 4% bovine serum albumin (BSA), pH7.4). The exposed gonads were then washed once in the staining buffer and transferred to a ringed slide (Fisher 22-339-408) coated with polylysine. The gonads were then stained with anti-FLAG M2 antibody (Sigma-Aldrich, Cat. No. F3165; 1:100 dilution) in the staining buffer at room temperature for 30 min. Following anti-FLAG antibody staining, gonads were washed three times with the staining buffer and then stained with fluorescein isothiocyanate (FITC)-conjugated goat anti-mouse antibody (Jackson ImmunoResearch, code No. 115-095-003; 1:100 dilution) at room temperature for 20 min and then washed three times with the staining buffer. After that, gonads were stained with Rhodanmin Red-X-conjugated mouse anti-FITC antibody (Jackson ImmunoResearch, code No. 200-292-037; 1:100 dilution) and 4 μM Hoechst 33342 at room temperature for 20 min and washed three times with the staining buffer. The stained gonads were visualized using a fluorescent Nomarski microscope. For immunostaining using fixed, permeabilized conditions, staining buffer was removed from the exposed gonads and replaced with the fixation buffer (PBS containing 1% formaldehyde, pH 7.4) at room temperature for 30 min in a humidified chamber. After the fixation buffer was removed, gonads were incubated with the PBS buffer at room temperature for 5 min, washed three times with the PBS buffer and then incubated in permeabilizing buffer (PBS containing 0.1% Triton-X-100 and 0.1% sodium citrate, pH 7.4) for 1 min. The permeabilized gonads were washed three times with the PBS buffer and incubated in staining buffer at room temperature for 30 min, before the addition of anti-Flag M2 antibody (1:100 dilution) at room temperature for 1 h. Staining with the FITC-conjugated goat anti-mouse antibody (1:100 dilution) and Rhodamine Red-X-conjugated mouse anti-FITC antibody (1:100 dilution) and visualization of stained gonads were performed as described above in non-permeabilized staining protocol, exception that staining time is 45 min each. To stain C. elegans embryos, mix-stage animals were harvested with the M9 buffer, bleached with 12% NaOCl and 1.5 M NaOH and centrifuged at 500 g to remove bacteria and debris. Embryos were washed three times with H 2 O, mounted on poly- L -lysine coated slides and frozen at −80 °C for 10 min. They were fixed with methanol for 15 min followed by 4% paraformaldehyde (Sigma) for 10 min on ice and washed with PBS before being stained with anti-Flag M2 antibody (1:100 dilution) in PBS for 1 h. Staining with the FITC-conjugated goat anti-mouse antibody (1:100 dilution) and Rhodamine Red-X-conjugated mouse anti-FITC antibody (1:100 dilution) in the presence of DAPI (Vector) and visualization of stained embryos were performed as described above in the permeabilized staining protocol. Co-immunoprecipitation assay in C. elegans smIs350 (P tra-2 TRA-2::3xFlag) animals or ced-1(e1735); smIs510 (3xflag::psr-1 SCI) ; psr-1(tm469) animals were cultured in liquid medium for 4 days, harvested and washed three times with 100 mM NaCl [59] . Bacteria and fungi were removed by sucrose gradient centrifugation. The animals were then lysed by sonication in the lysis buffer (20 mM HEPES, 100 mM NaCl, 0.5% (v/v) NP-40 and 1 mM EDTA) with protease inhibitors. Supernatant was collected through centrifugation at 14,000 g at 4 °C for 30 min, precleared with Protein G beads (GE Healthcare) and then incubated for 2 h with the anti-Flag M2 affinity gel (Sigma-Aldrich) at 4 °C with gentle shaking. After four washes with the same buffer, the samples were resolved on 12.5% SDS–polyacrylamide gels, transferred to a PVDF membrane and detected by immunoblotting using mouse anti-Flag M2 antibody (Sigma-Aldrich, Cat. No. F3165; 1:5,000 dilution) and horseradish peroxidase (HRP)-conjugated goat anti-mouse light-chain-specific antibodies (Jackson ImmunoResearch, code No. 115-035-174; 1:10,000 dilution) or rabbit anti-CED-2 antibodies (Novus Biologicals, Cat. No. 42090002; 1:1,000 dilution for co-IP samples and 1:5,000 for lysates) and HRP-conjugated goat anti-rabbit antibodies (BIO-RAD, Cat. No. 170-6515; 1:20,000 dilution). Purification of proteins The fragments of C. elegans PSR-1 cDNA (corresponding to residues 293–400, 293–349, 293–320 and 321–400, respectively), the fragment of human PSR (hPSR) cDNA (corresponding to residues 288–403) or the fragment of Lactadherin cDNA (corresponding to residues 306–464) were subcloned into the pET-41b vector through its SpeI and XhoI sites to generate constructs expressing GST-tagged fusion proteins. The GST fusion protein was expressed in E. coli strain BL21 through the induction by 0.5 mM isopropyl-β- D -thiogalactopyranoside when the cell density reached an OD 600 nm of 0.8. After growth at 23 °C for 7 h, the cells were harvested, resuspended in lysis buffer (1 × PBS, 2 mM DTT and 1 mM PMSF) and lysed using sonication. The cell lysate was centrifuged at 20,000 g for 45 min at 4 °C to remove cell debris. The cleared supernatant was applied onto a GST-affinity column (2 ml glutathione Sepharose 4B; GE Healthcare) and contaminant proteins were removed with wash buffer (lysis buffer with 200 mM NaCl). The GST fusion protein was then eluted with elution buffer (50 mM Tris-HCl pH 7.5, 200 mM NaCl, and 20 mM reduced glutathione). The eluted protein was concentrated using an Ultrafree 10000 molecular-weight cutoff filter unit (Millipore) and further purified using a Superdex-200 column (GE Healthcare) equilibrating with a buffer containing 10 mM Tris-HCl pH 8.0, 200 mM NaCl and 2 mM DTT. The purified fusion protein was then analysed by 15% SDS–PAGE. The fractions containing the GST fusion protein were pooled and stored at −80 °C. The fragments of C. elegans PSR-1 cDNA (corresponding to residues 1–270 and residues 293–400) were subcloned into a modified pET-15b vector with a MBP tag through its NdeI and XhoI sites to generate constructs expressing His 6 -MBP tagged fusion proteins. The expression of the His 6 -MBP fusion protein was induced similarly as that used for the GST fusion proteins described above. The His 6 -MBP fusion protein was first purified using Ni 2+ -affinity chromatography and then size-exclusion chromatography (Superdex-200 column) with buffer (10 mM Tris-HCl pH 8.0, 200 mM NaCl, 2 mM DTT) on a FPLC system (GE Healthcare Life Sciences). Lipid-binding assays The membrane lipid strips were made using the standard method [60] . In brief, we spotted 500 pmol of each phospholipid (Avanti Polar Lipids) onto Hybond-C extra membrane (GE Healthcare Life Sciences) and allowed the membrane strips to dry at room temperature for 1.5 h. The membrane strips were then blocked with 5% (w/v) fatty acid-free BSA in PBST buffer (PBS with 0.01% tween 20 and 0.5 mM CaCl 2 ) for 1.5 h and incubated with 5 μg ml −1 GST or His 6 -MBP fusion protein in the same blocking buffer at 4 °C overnight. After washing the membrane strips three times for 10 min each with 0.5% (w/v) fatty acid-free BSA in PBST (PBS with 0.05% tween 20 and 0.5 mM CaCl 2 ), the membrane strips were incubated with anti-GST or anti-His 6 polyclonal antibodies for 2 h. The membrane strips were washed as above with 0.5% (w/v) fatty acid-free BSA in PBST (PBS with 0.05% tween 20 and 0.5 mM CaCl 2 ) and incubated for 1 h with HRP-conjugated anti-rabbit antibody (Kirkegaard & Perry Laboratories, Cat. No. 474–1506; 1:5,000 dilution). After washing the membrane strips with 0.5% (w/v) fatty acid-free BSA in PBST (PBS with 0.05% tween 20 and 0.5 mM CaCl 2 ) five times each for 10 min, the proteins bound to the membrane strip were detected by the ECL detection reagents. Preparation of liposomes Liposomes were prepared following established protocols [61] . In brief, the synthetic lipids (Avanti Polar Lipids) were mixed in chloroform, dried under N 2 and vacuum dried overnight before resuspension in HEPES buffered saline with Ca 2+ (10 mM HEPES, 0.15 mM NaCl and 2 mM CaCl 2 ). Resuspended lipids were freeze-thawed five times and extruded nine times through 0.8 μm pore size filters (Whatman). Liposome models tested were: PC liposomes (67.5% PC, 16% Cholesterol, 16.5% Sphingomyelin); PS liposomes (57.5% PC, 10% PS, 16% Cholesterol, 16.5% Sphingomyelin); PA liposomes (57.5% PC, 10% PA, 16% Cholesterol, 16.5% Sphingomyelin); PE liposomes (57.5% PC, 10% PE, 16% Cholesterol, 16.5% Sphingomyelin); PI liposomes (57.5% PC, 10% Soy PI, 16% Cholesterol, 16.5% Sphingomyelin). Tryptophan fluorescence quenching assays Fluorescence measurements were performed on a Fluorolog-3 spectrofluorimeter (Horiba Jobin Yvon, Edison, NJ, USA). All measurements were carried out under room temperature in a 2 × 10 mm quartz cell (Starna Cells, Atascadero, CA, USA). An excitation wavelength of 295 nm was chosen and emission at 310–450 nm was measured. PSR-1 proteins (0.2 μΜ) were titrated with different concentrations of liposomes, and the fluorescence intensity at 340 nm was plotted against liposomes concentration. The raw data were fitted by non-linear least square method using the equation: F =0.5 × (2 × F 0 − F PL × ( K D +[ L T ]+[ P T ]−(( K D +[ L T ]+[ P T ]) 2 −4 × [ L T ] × [ P T ]) 0.5 )), where [ F ], the observed fluorescence; F 0 , the initial fluorescence of protein in the absence of liposome; F PL , adjustable parameter for protein–liposome complex molar fluorescence; K D , dissociation constant; [ L T ], the total concentration of the liposome; [ P T ], total protein concentration. Size-exclusion chromatography Size-exclusion chromatography was performed using a Superdex-200 column equilibrated with a modified PBS buffer with 2 mM DTT, 0.5 mM CaCl 2 and 200 mM NaCl. The protein sample (1 mg ml −1 ) was applied to the column in a total volume of 1 ml after incubating with 400 μg ml −1 of phospholipid (dissolved in 0.08% DM) or 0.08% DM at 4 °C for 1 h, and the flow-through fractions were collected and analysed by 15% SDS–PAGE. Crosslinking of PSR-1 proteins Proteins from Superdex-200 flow-through fractions were incubated on ice with 25 μM BS3 crosslinker (Thermo Scientific) in a modified PBS buffer with 2 mM DTT, 0.5 mM CaCl 2 , 200 mM NaCl and 0.08% DM for 60 min. The reactions were terminated using 50 mM glycine, resolved on 8% SDS–PAGE and then transferred to the PVDF membrane (Millipore). The membrane strips were blocked with 5% (W/V) BSA in TBST buffer (50 mM Tris-HCl pH 7.4, 150 mM NaCl and 0.05% Tween 20) and then incubated with anti-His 6 monoclonal antibody (ProteinTech, Cat. No. 66005-1-Ig; 1:5,000 dilution) to detect C-terminally His-tagged PSR-1 proteins. Statistical analysis If not stated otherwise, results are presented as mean±s.e.m. The significance of difference between two strains was compared by Student’s t -test. How to cite this article: Yang, H. et al. A lysine-rich motif in the phosphatidylserine receptor PSR-1 mediates recognition and removal of apoptotic cells. Nat. Commun. 6:5717 doi: 10.1038/ncomms6717 (2015).